HuR and miR-1192 regulate myogenesis by modulating the translation ofHMGB1mRNA Upon muscle injury, the high mobility group box 1 (HMGB1) protein is upregulated and secreted to initiate reparative responses. Here we show that HMGB1 controls myogenesis both in vitro and in vivo during development and after adult muscle injury. HMGB1 expression in muscle cells is regulated at the translational level: the miRNA miR-1192 inhibits HMGB1 translation and the RNA-binding protein HuR promotes it. HuR binds to a cis -element, HuR binding sites (HuRBS), located in the 3′UTR of the HMGB1 transcript, and at the same time miR-1192 is recruited to an adjacent seed element. The binding of HuR to the HuRBS prevents the recruitment of Argonaute 2 (Ago2), overriding miR-1192-mediated translation inhibition. Depleting HuR reduces myoblast fusion and silencing miR-1192 re-establishes the fusion potential of HuR-depleted cells. We propose that HuR promotes the commitment of myoblasts to myogenesis by enhancing the translation of HMGB1 and suppressing the translation inhibition mediated by miR-1192. The process leading to muscle fibre formation during embryonic development, also known as myogenesis, involves the fusion of mononucleated myoblasts to form multinucleated myofibers [1] . Likewise, upon injury, adult muscle tissues are repaired by satellite cells, which are quiescent mononucleated cells that coexist with myofibers [2] . In response to injuries, satellite cells are activated; they first proliferate and then exit the cell cycle to fuse and form muscle fibre [3] , [4] , [5] . During both embryonic and injury-induced myogenesis, a cohort of intra- and extra-cellular factors act in concert. HMGB1 (the high mobility group box 1) is a cytokine that is secreted by damaged muscle fibres and by infiltrating inflammatory cells after muscle injury. One of its main functions is to promote myogenesis by associating with the receptor for advanced glycation end products, which is expressed on the surface of myoblasts, resulting in the activation of a signal transduction cascade that induces the expression of promyogenic factors such as MyoD and myogenin [6] , [7] , [8] , [9] , [10] , [11] , [12] . It is also known that while HMGB1 is highly expressed in myoblasts or satellite cells, its level in muscle fibres is significantly reduced [3] , [9] . This suggests that maintaining a high expression level of HMGB1 during the early steps of myogenesis is required for the formation of functional myotubes. However, the mechanism controlling HMGB1 levels during myogenesis have never been investigated. It has been shown that the 3′ untranslated region (3′UTR) of HMGB1 messenger RNA (mRNA) is very long and contains elements that are uridyl-rich (U-rich) [13] . U-rich elements in the 3′UTR are known to modulate posttranscriptional events such as the cellular movement, the turnover and the translation of many mRNAs [14] , [15] . The expression of mRNAs encoding MyoD and myogenin is regulated posttranscriptionally. These mRNAs harbour AU-rich elements located in their 3′UTRs that mediate their association with RNA-binding proteins such as HuR. This association is crucial for the stability and the expression of these messages during myogenesis [16] , [17] . As HuR binds to MyoD and myogenin mRNAs only during the transition state from myoblasts to myotubes but not at earlier stages [17] , we concluded that HuR promotes myogenesis by stabilizing these mRNAs specifically at this later step during the myogenic process. However, knocking down the expression of HuR in undifferentiated muscle cells prevented their entry into the differentiation process [17] . Thus, HuR-dependent promyogenic activities could also involve modulating the expression of mRNA targets during the early steps of myogenesis. In this study, we show that HMGB1 is required for myogenesis and that its expression in muscle cells is controlled at the translational level. Both miR-1192 and HuR associate with a U-rich element in the 3′UTR of the HMGB1 mRNA. miR-1192 inhibits HMGB1 translation, but HuR promotes the translation of HMGB1 mRNA by preventing the formation of Argonaute 2 (Ago2)/miR-1192 complex. We propose that HuR promotes the commitment of myoblasts to myogenesis by enhancing the translation of HMGB1 and suppressing the translation inhibition mediated by miR-1192. The HuR-mediated expression of HMGB1 promotes myogenesis HuR modulates the expression of MyoD and myogenin mRNAs in an ARE-dependent manner during the transition state from myoblasts to myotubes, but not at the earlier stages [16] , [17] , [18] . To identify potential HuR mRNA targets during the early steps of myogenesis, we performed an immunoprecipitation (IP) experiment combined with cDNA microarray analysis on total extracts from undifferentiated C2C12 cells, a well-established murine myogenic cell line [19] . C2C12 cell extracts were immunoprecipitated with an anti-HuR or –immunoglobulin G (IgG) antibody. The RNAs associated with HuR were isolated and hybridized to mouse arrays. We revealed that HuR bound to 64 mRNAs in undifferentiated myoblasts ( Supplementary Table S1 ). Among these messages, HMGB1 and the β -actin mRNAs are known to encode proteins that directly affect muscle cell differentiation [9] , [10] , [20] . As HuR associates with MyoD and myogenin mRNAs only at later stages of the myogenic process [17] , [21] , these messages were not on this list. While β-actin mRNA expression is known to depend on HuR [22] , nothing is known regarding the link between HMGB1 expression, its promyogenic function and HuR protein. Using IP coupled with quantitative (q) reverse transcriptase–PCR (RT–qPCR), we validated the association between HuR and HMGB1 mRNA in these cells ( Supplementary Fig. S1a,b ). Therefore, it is possible that HuR regulates HMGB1 expression during the early steps of myogenesis. Several studies have suggested that the high expression level of HMGB1 in myoblasts is important for myogenesis [3] , [9] . Indeed, we observed that while HMGB1 mRNA and protein are highly expressed during the early steps of muscle cell differentiation, their expression decreases at later steps ( Supplementary Fig. S2 ). Despite this, the role of HMGB1 in the commitment of muscle cells to myogenesis is still elusive. To address this question, we depleted the expression of HMGB1 or HuR in C2C12 cells and the efficiency of myogenesis was determined by assessing cell morphology by phase contrast, the expression of the Myosin heavy chain (My-HC) by immunofluorescence (IF), and by determining the fusion index [17] ( Fig. 1a–e ). We observed that HMGB1 depletion reduced the efficiency of muscle fibre formation by >85% ( Fig. 1c–e ). As expected [17] , a similar reduction in myogenesis was also observed in C2C12 depleted of HuR. Western blot analysis showed that the levels of My-HC and to a lesser extent myoglobin were reduced due to the knockdown of HMGB1 or HuR ( Fig. 1f ). Interestingly, exposing C2C12 cells depleted of endogenous HMGB1 to 400 nM of recombinant HMGB1 (rHMGB1) re-established their ability to enter the myogenic process ( Supplementary Fig. S2c,d ). These observations demonstrate that HMGB1 promotes the early steps of myogenesis via its extracellular association with the receptor for advanced glycation end products. 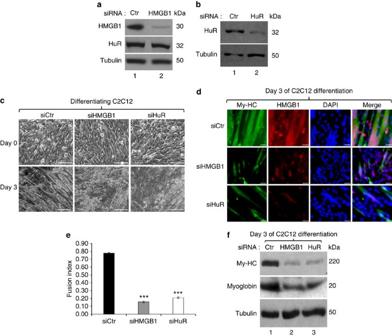Figure 1: Knocking down HMGB1 expression in myoblasts prevents their entry into the myogenic process. (a,b) HuR and HMGB1 knockdown were performed in C2C12 cells and total cell lysates were prepared 48 h post-transfection. Western blotting was performed using antibodies against HMGB1, HuR and α-tubulin as a loading control. (c) Phase contrast pictures showing the morphology of C2C12 cells transfected with control (siCtr), siHMGB1 or siHuR, at the time of differentiation induction (day 0) and at day 3. Scale bars, 50 μm(d) IF with anti-My-HC, anti-HMGB1 antibodies and DAPI was performed to determine the differentiation status of the C2C12 cells treated with the indicated siRNAs. Scale bars, 20 μm. Representative images from three independent experiments are shown. (e) The fusion index indicating the efficiency of C2C12 differentiation was determined by calculating the number of nuclei in cells with more than 2 nuclei (myotubes) in relation to the total number of nuclei in each microscopic field. Data are presented as +/− s.e.m. of three independent experiments. ***P<0.0001 (t-test). (f) Total cell extracts were prepared at day 3 of differentiation. Western blotting was performed using antibodies against My-HC, myoglobin, and α-tubulin as a loading control. Blots shown in a–b–f are representative of three independent experiments. Figure 1: Knocking down HMGB1 expression in myoblasts prevents their entry into the myogenic process. ( a , b ) HuR and HMGB1 knockdown were performed in C2C12 cells and total cell lysates were prepared 48 h post-transfection. Western blotting was performed using antibodies against HMGB1, HuR and α-tubulin as a loading control. ( c ) Phase contrast pictures showing the morphology of C2C12 cells transfected with control (siCtr), siHMGB1 or siHuR, at the time of differentiation induction (day 0) and at day 3. Scale bars, 50 μ m ( d ) IF with anti-My-HC, anti-HMGB1 antibodies and DAPI was performed to determine the differentiation status of the C2C12 cells treated with the indicated siRNAs. Scale bars, 20 μm. Representative images from three independent experiments are shown. ( e ) The fusion index indicating the efficiency of C2C12 differentiation was determined by calculating the number of nuclei in cells with more than 2 nuclei (myotubes) in relation to the total number of nuclei in each microscopic field. Data are presented as +/− s.e.m. of three independent experiments. *** P <0.0001 ( t- test). ( f ) Total cell extracts were prepared at day 3 of differentiation. Western blotting was performed using antibodies against My-HC, myoglobin, and α-tubulin as a loading control. Blots shown in a–b–f are representative of three independent experiments. Full size image Next, we assessed the impact of HMGB1 on muscle development and growth in vivo using Hmgb1 wild-type (wt) (+/+), +/− and −/− mice. During vertebrate embryogenesis, skeletal muscle in the limb develops from progenitor cells originating in the somites [23] . Mice where the Hmgb1 gene has been deleted die perinatally [24] . To assess the role of HMGB1 in mouse myogenesis, we therefore crossed Hmgb1 +/− mice with homozygous MLC1/3F-nlacZ transgenic mice (wt for Hmgb1 ) [25] and collected the embryos at E10.5. As expected, half of the embryos were Hmgb1 +/+ , whereas the other half was Hmgb1 +/− ; all of them carried the MLC1/3F-nlacZ transgene and showed blue myonuclei when stained for X-gal ( Fig. 2 ). We observed a significant reduction in the number of somites in Hmgb1 +/− embryos when compared with wt controls ( Fig. 2a ). We then collected explants from wt, Hmgb1 +/− and Hmgb1 −/− embryos (E9.5), cultured them for 4 days [26] and determined the differentiation efficiency of myoblasts. We observed that Hmgb1 −/− and +/− myoblasts formed significantly fewer myotubes than wt myoblasts ( Fig. 2b ). We next analysed 1-year-old Hmgb1 +/− mice to score for any reduction in muscle mass and cellularity when compared with wt mice. Hmgb1 +/− mice showed a significant reduction in both total body weight and the mass of the tibialis anterior (TA) muscle ( Fig. 2c ). The myofibers in the TA muscle of Hmgb1 +/− mice had a smaller cross-sectional area (XSA) than those of control mice ( Fig. 2d,e ). We also confirmed that mouse embryonic fibroblasts and muscle tissue from Hmgb1 +/− mice express 50% less HMGB1 than their Hmgb1 +/+ counterparts ( Fig. 2f ). Additionally, a muscle injury experiment showed a marked delay in the Hmgb1 +/− mice in the regeneration process after injury as evidenced by the significant reduction in the XSA of regenerating fibres at both 7 and 14 days after injury ( Fig. 3 ). 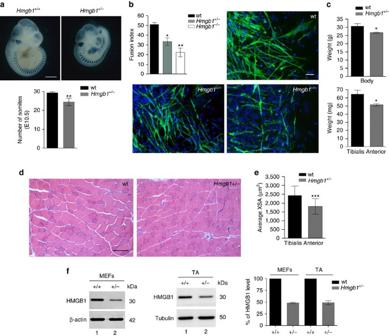Figure 2: HMGB1 is required for proper muscle fibre formationin vivo. (a) Top panel: whole-mount X-Gal staining of control heterozygote MLC1/3 F-nlacZ and double heterozygote MLC1/3 F-nlacZ-Hmgb1+/−embryos collected at E10.5. Scale Bars, 1 mm. Bottom panel: Histogram showing the average number of somites expressing MLC1/3 F-nlacZ in control and double heterozygotes embryos at E10.5. **P<0.01 indicates a significant reduction in the number of transgene-expressing somites inHmgb1+/−embryos compared withHmgb1+/+(Data are presented as +/− s.d.,t-test,n=6). (b) PSM explants were derived from wt,Hmgb1+/−andHmgb1−/−embryos (E9.5), cultured for 4 days and analysed by IF with a specific antibody against My-HC (green) and DAPI counterstaining (blue). Scale bar, 20 μm. Fusion index was calculated as the number of nuclei in My-HC positive cells with more than 2 nuclei (myotubes) in relation to the total number of nuclei in each microscopic field. Data are presented as +/− s.d. of three independent experiments. *P<0.05 and **P<0.01 (t-test,n=3). (c) Body and TA weights of 1-year-old wt andHmgb1+/−mice. Three animals were analysed per group. Error bars represent s.d. *P<0.05 (t-test). (d) Histology of TA muscle. Representative images of H&E stained sections of TA muscles of 3-month-old wt andHmgb1+/−mice. Scale bar, 100 μm. (e) Mean cross-section area (XSA) of TA muscle fibres from 1-year-old wt andHmgb1+/−mice. Error bars represent s.d. Nine hundred fibres were analysed for each group. ***P<0.001 versus wt (analysis of variance). (f) Western blots for HMGB1 were performed on equal amounts of total extracts from wt (+/+) and heterozygous (+/−) MEFs and adult TA. β-actin and tubulin are shown as loading controls. The blots shown are representative of three independent experiments. Western blot signals were quantified with ImageQuant software (GE Healthcare) and plotted +/− s.d. from three independent experiments. Figure 2: HMGB1 is required for proper muscle fibre formation in vivo . ( a ) Top panel: whole-mount X-Gal staining of control heterozygote MLC1/3 F-nlacZ and double heterozygote MLC1/3 F-nlacZ- Hmgb1+/− embryos collected at E10.5. Scale Bars, 1 mm. Bottom panel: Histogram showing the average number of somites expressing MLC1/3 F-nlacZ in control and double heterozygotes embryos at E10.5. ** P <0.01 indicates a significant reduction in the number of transgene-expressing somites in Hmgb1+/− embryos compared with Hmgb1+/+ (Data are presented as +/− s.d., t -test, n =6). ( b ) PSM explants were derived from wt, Hmgb1+/− and Hmgb1−/− embryos (E9.5), cultured for 4 days and analysed by IF with a specific antibody against My-HC (green) and DAPI counterstaining (blue). Scale bar, 20 μm. Fusion index was calculated as the number of nuclei in My-HC positive cells with more than 2 nuclei (myotubes) in relation to the total number of nuclei in each microscopic field. Data are presented as +/− s.d. of three independent experiments. * P <0.05 and ** P <0.01 ( t -test, n =3). ( c ) Body and TA weights of 1-year-old wt and Hmgb1+/− mice. Three animals were analysed per group. Error bars represent s.d. * P <0.05 ( t -test). ( d ) Histology of TA muscle. Representative images of H&E stained sections of TA muscles of 3-month-old wt and Hmgb1+/− mice. Scale bar, 100 μm. ( e ) Mean cross-section area (XSA) of TA muscle fibres from 1-year-old wt and Hmgb1+/− mice. Error bars represent s.d. Nine hundred fibres were analysed for each group. *** P <0.001 versus wt (analysis of variance). ( f ) Western blots for HMGB1 were performed on equal amounts of total extracts from wt (+/+) and heterozygous (+/−) MEFs and adult TA. β-actin and tubulin are shown as loading controls. The blots shown are representative of three independent experiments. Western blot signals were quantified with ImageQuant software (GE Healthcare) and plotted +/− s.d. from three independent experiments. 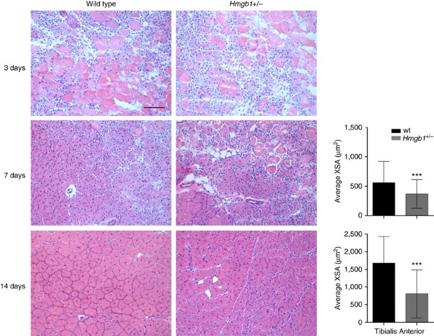Figure 3: HMGB1 is required for normal muscle regeneration after injury. Representative sections of TA muscles from wt andHmgb1+/− mice stained with H&E 3, 7 and 14 days after CTX injury. Scale bar, 100 μm. The cross-sectional area (XSA) of regenerating TA myofibers was decreased inHmgb1+/−mice at both 7 and 14 days following injury. Nine hundred fibres were analysed for each group (three animals per group). Error bars in the histograms represent s.d. ***P<0.001 versus wt (analysis of variance). Full size image Figure 3: HMGB1 is required for normal muscle regeneration after injury. Representative sections of TA muscles from wt and Hmgb1 +/− mice stained with H&E 3, 7 and 14 days after CTX injury. Scale bar, 100 μm. The cross-sectional area (XSA) of regenerating TA myofibers was decreased in Hmgb1+/− mice at both 7 and 14 days following injury. Nine hundred fibres were analysed for each group (three animals per group). Error bars in the histograms represent s.d. *** P <0.001 versus wt (analysis of variance). Full size image Together, these data demonstrate that maintaining a high expression level of HMGB1 in myoblasts is required for embryonal myogenesis and muscle regeneration after acute injury because of its release from myoblasts and/or damaged myofibers [10] , [12] , [27] . HuR promotes the translation of the HMGB1 mRNA The HuR protein is known to modulate the export, stability and/or the translation of its target mRNAs [14] , [28] . The fact that HuR has a key role during the early steps of myogenesis [17] and associates with HMGB1 mRNA in muscle cells ( Supplementary Fig. S1 ) suggested that HuR promotes muscle differentiation by regulating HMGB1 expression posttranscriptionally. Hence, we first determined whether HuR is required for the expression of HMGB1 in C2C12 cells. We observed that knocking down HuR in myoblasts reduced the levels of the HMGB1 protein (by >65%), but not its three mRNA isoforms ( Fig. 4a–d ). Pulse-chase mRNA stability experiments [22] , RNA fluorescence in situ hybridization [29] and cellular fractionation indicated that HuR does not affect the cellular movement or the stability of HMGB1 messages ( Supplementary Figs. S3 and 4 ). These observations therefore suggest that HuR regulates the translation of the HMGB1 mRNA. Sucrose fractionation experiments were performed to assess this possibility. We observed that while the depletion of HuR had no significant effect on the general distribution profile of polysomes ( Fig. 4e ), knocking down HuR resulted in a shift in the distribution of HMGB1 mRNA towards lighter polysome fractions when compared with siCtr-treated cells. These results indicated that the HMGB1 transcript is less translated in the absence of HuR ( Fig. 4f ). As HuR-mediated effects on target mRNAs in muscle cells have been linked to its ability to accumulate in the cytoplasm [30] , we tested whether this could also be the case for HMGB1 mRNA. To do this, we treated undifferentiated C2C12 cells with the HuR cleavage product 1 (HuR-CP1), which promotes the cytoplasmic accumulation of HuR during myogenesis [30] . We observed that HuR-CP1 increased HuR level in the cytoplasm of muscle cells and promoted the expression of the HMGB1 protein ( Fig. 4g,h ). Taken together, these results show that HuR maintains the high expression level of HMGB1 in muscle cells by promoting the translation of HMGB1 mRNA. 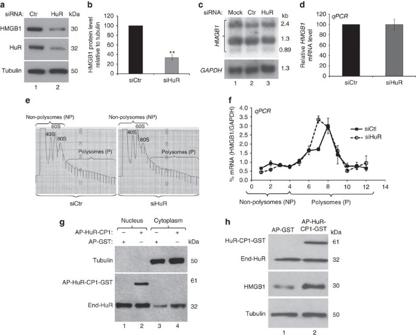Figure 4: HuR promotes the translation of HMGB1 in C2C12 cells. (a) Total extracts from C2C12 cells treated with siHuR or siCtr were used for western blots with antibodies against HMGB1, HuR and α-tubulin as a loading control. (b) The HMGB1 protein level relative to α-tubulin for each treatment was plotted as the percentage relative to siCtr-treated sample +/− the s.e.m. of three independent experiments. **P<0.001 (t-test). (c) Northern blot of total RNA from C2C12 cells treated with siHuR or siCtr. A representative blot of three independent experiments is shown. (d) Total RNAs from siHuR- or siCtr-treated C2C12 cells were subjected to RT–qPCR analysis using specific primers forHMGB1andGAPDHmRNAs and plotted +/− the s.e.m from three independent experiments. (e) Sucrose gradient (15–50%) polysome fractionation of extracts from exponentially growing C2C12 cells that were treated with siHuR or siCtr. The profile of polysome distribution did not differ between C2C12 cells treated with siHuR or siCtr. (f) Quantitative RT–PCR was performed on the sucrose fractions using specific primers forHMGB1andGAPDHmRNAs. Error bars represent s.e.m. from four independent experiments. (g,h) C2C12 cells were treated with HuR-CP1 as described30. The nuclear and cytoplasmic fractions (g) or total extracts (h) were prepared and used for western blot analysis with anti-HuR, -HMGB1 and α-tubulin antibodies. All blots shown ingandhare representative of three independent experiments. Figure 4: HuR promotes the translation of HMGB1 in C2C12 cells. ( a ) Total extracts from C2C12 cells treated with siHuR or siCtr were used for western blots with antibodies against HMGB1, HuR and α-tubulin as a loading control. ( b ) The HMGB1 protein level relative to α-tubulin for each treatment was plotted as the percentage relative to siCtr-treated sample +/− the s.e.m. of three independent experiments. ** P <0.001 ( t -test). ( c ) Northern blot of total RNA from C2C12 cells treated with siHuR or siCtr. A representative blot of three independent experiments is shown. ( d ) Total RNAs from siHuR- or siCtr-treated C2C12 cells were subjected to RT–qPCR analysis using specific primers for HMGB1 and GAPDH mRNAs and plotted +/− the s.e.m from three independent experiments. ( e ) Sucrose gradient (15–50%) polysome fractionation of extracts from exponentially growing C2C12 cells that were treated with siHuR or siCtr. The profile of polysome distribution did not differ between C2C12 cells treated with siHuR or siCtr. ( f ) Quantitative RT–PCR was performed on the sucrose fractions using specific primers for HMGB1 and GAPDH mRNAs. Error bars represent s.e.m. from four independent experiments. ( g , h ) C2C12 cells were treated with HuR-CP1 as described [30] . The nuclear and cytoplasmic fractions ( g ) or total extracts ( h ) were prepared and used for western blot analysis with anti-HuR, -HMGB1 and α-tubulin antibodies. All blots shown in g and h are representative of three independent experiments. Full size image HuR prevents miR-1192-mediated repression of HMGB1 translation HuR affects the translation of target messages by associating with HuRBS located at either the 5′ or 3′UTRs [14] . Sequence analysis revealed the presence of a U-rich element in the 3′UTR of the HMGB1 mRNA that is similar to a HuRBS in the β-actin mRNA [22] ( Fig. 5a ). To assess whether this and/or other elements could mediate HuR binding, we performed RNA electromobility shift assays using total extracts from C2C12 cells and thirteen radiolabelled cRNA probes that covered the entire 5′ and 3′ UTRs of HMGB1 mRNA ( Fig. 5a ). All the probes except P6 and P8 formed RNA-protein complexes when incubated with total cell extract ( Fig. 5b ). However, an anti-HuR antibody only shifted RNA-complexes (HuR-C) containing the P4 but not the other probes ( Fig. 5b ). A pull-down experiment confirmed the specificity of HuR binding: biotinylated P4 associated with HuR but not with CUGBP1, an RNA-binding protein known to modulate muscle differentiation [31] ( Supplementary Fig. S5a ). 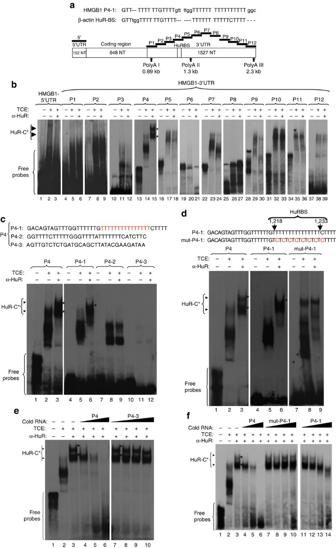Figure 5: HuR specifically binds to a U-rich element within theHMGB13′UTR. (a) Upper panel: alignment of the U-rich HuRBS within theHMGB1and β-actin3′UTRs. Lower panel: schematic representation of theHMGB1mRNA sequence. The elements covering the 5′ and the 3′ (P1-P12) UTRs ofHMGB1used to generate radiolabelled RNA probes for RNA electromobility shift assays are indicated. The accession number in the NCBI database of theHMGB1mRNA sequence used to generate these probes is NM_010439. (b–f) Representative gels of supershifts carried out by incubating C2C12 TCE with radiolabelled cRNA probes and anti-HuR antibody. Supershifted complexes (HuR-C) contain HuR protein. (b) Gel-shift assay performed using radiolabelled 5′UTR and the 12 probes (P1 to P12) depicted in (a). (c) Nucleotide sequence of the probes P4-1, P4-2 and P4-3 that were generated to localize HuR binding site (upper panel). These probes were used for gel-shift assays (lower panel). (d) Nucleotide sequences of probe P4-1 (HuRBS) and mut-P4-1, showing the T->C changes in mut-P4-1 (upper panel). The arrowhead shows HuR-C (lower panel). (e,f) Gel-shift competition was performed with radiolabelled probe P4 and 1 × , 10 × and 100 × excess of the indicated unlabelled probes. All blots shown inb–fare representative of three independent experiments. Figure 5: HuR specifically binds to a U-rich element within the HMGB1 3′UTR. ( a ) Upper panel: alignment of the U-rich HuRBS within the HMGB1 and β -actin 3′UTRs. Lower panel: schematic representation of the HMGB1 mRNA sequence. The elements covering the 5′ and the 3′ (P1-P12) UTRs of HMGB1 used to generate radiolabelled RNA probes for RNA electromobility shift assays are indicated. The accession number in the NCBI database of the HMGB1 mRNA sequence used to generate these probes is NM_010439. ( b – f ) Representative gels of supershifts carried out by incubating C2C12 TCE with radiolabelled cRNA probes and anti-HuR antibody. Supershifted complexes (HuR-C) contain HuR protein. ( b ) Gel-shift assay performed using radiolabelled 5′UTR and the 12 probes (P1 to P12) depicted in ( a ). ( c ) Nucleotide sequence of the probes P4-1, P4-2 and P4-3 that were generated to localize HuR binding site (upper panel). These probes were used for gel-shift assays (lower panel). ( d ) Nucleotide sequences of probe P4-1 (HuRBS) and mut-P4-1, showing the T->C changes in mut-P4-1 (upper panel). The arrowhead shows HuR-C (lower panel). ( e , f ) Gel-shift competition was performed with radiolabelled probe P4 and 1 × , 10 × and 100 × excess of the indicated unlabelled probes. All blots shown in b–f are representative of three independent experiments. Full size image To delineate the HuRBS within P4, we divided this element into radiolabelled cRNA probes P4-1, -2 and -3 ( Fig. 5c ). A supershift containing the HuR-C was only generated with P4-1. A P4-1 mutant probe (mut-P4-1) in which every second U in the U-rich element (U 15 ) was changed to a C ( Fig. 5d ) also failed to form a complex when incubated with extracts in the presence of the anti-HuR antibody. P4-HuR complexes were gradually competed away in the presence of an excess of unlabelled P-4 or P4-1 probes but not in the presence of an excess of unlabelled P4-3 or mut-P4-1 probes ( Fig. 5e,f ). These observations, together with the fact that recombinant GST-HuR but not GST alone was able to form an HuR-C ( Supplementary Fig. S5b ), demonstrate that the U 15 element located between nucleotides (nt) 1218 and 1233 comprises the HuRBS in the HMGB1 -3′UTR. Previous studies have indicated that HuR either competes or collaborates with miRNAs in order to regulate the translation of some of its mRNA targets [32] , [33] . We investigated whether this could also be the case for HMGB1 expression in muscle cells. As a first step, we identified miRNAs that associate with HuR in muscle cells. C2C12 cell extracts were immunoprecipitated with an anti-HuR antibody as described above and the miRNAs associated with HuR were isolated and identified using miRNA arrays (Exiqon, USA). We identified 20 miRNAs that were immunoprecipitated twofolds or more with the anti-HuR antibody when compared with the IgG control ( Supplementary Table S2 ). Using the MSKCC ( http://www.microrna.org/microrna/releaseNotes.do ), the BiBiSer ( http://bibiserv.techfak.uni-bielefeld.de/rnahybrid/ ) and the miRmap ( http://mirmap.ezlab.org/app/ ) websites, we identified that among these 20 HuR-miRNAs only miR-1192 is predicted to target the HMGB1 mRNA. miR-1192 stood out, as the first seven Us (nt 1218-1225) of its ‘seed’ sequence (miRNA binding site, miRBS) are part of the U-rich element containing the HuRBS ( Fig. 6a,b ). Additionally, our screening (RT–qPCR and sequencing) indicated that miR-1192 is expressed in C2C12 cells as well as in muscle and heart tissues, but not in the lung, spleen, MEFs or HeLa cells ( Supplementary Fig. S6 and Supplementary Table S3 ). Therefore, it was possible that this miRNA could contribute to the modulation of HMGB1 expression in muscle cells. 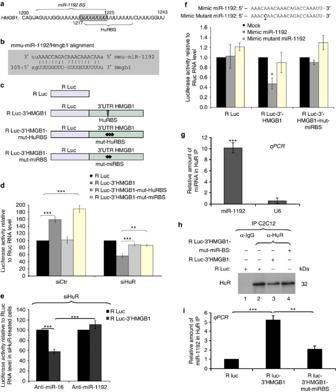Figure 6: HuR binding to a U8 element within HuRBS is sufficient to prevent the miR-1192-mediated inhibition of HMGB1 translation. (a) Schematic representation of the HuRBS and the seed element of miR-1192 (miR-1192 BS). (b) Diagram illustrating the bioinformatic approach used to predict miR-1192 as a putative miRNA targetingHMGB13′UTR. Shown here are complementarities of miR-1192 withHMGB13′UTR. (c) Schematic diagrams of luciferase constructs. (d–g) Effects of HuR, miRNAs, antagomirs and mimics. Error bars represent s.e.m of three independent experiments. ***P<0.0001, **P<0.001, *P<0.05 (Student’st-test). The amount of reporter RNA expressed in cells was determined by qPCR and used to normalize R Luc activities for each treatment. (d) Exponentially growing C2C12 cells were treated with siCtr or siHuR and 24 h later luciferase constructs were introduced. Luciferase activity of R Luc construct was considered as 100%. (e) miR-1192 and miR-16 antagomirs were transfected in siHuR-treated C2C12 cells previously transfected either with R luc alone or R luc-3′HMGB1. (f) Upper panel: schematic representation of the Mimic miR-1192 and Mimic mutant miR-1192. The asterisk (*) indicates thea–cmutation in the Mimic mutant miR-1192. Lower panel: HeLa cells were transfected with Mimic miR-1192 or Mimic mutant miR-1192 and 24 h later luciferase constructs were transfected. The luciferase activity of the mock-treated cells was set as reference. (g) Immunoprecipitation experiments were performed using a monoclonal HuR antibody, or IgG as a control, on total cell lysates from exponentially growing C2C12 cells. RNA was isolated from the immunoprecipitate, and quantitative RT–PCR was performed using primers specific to miR-1192, miR-16 and U6 RNAs. The levels of miR-1192 and U6 RNAs in each IP were normalized against the level of miR-16. Error bars represent s.e.m of three independent experiments.T-test was used for statistical analysis. (h,i) Immunoprecipitation experiments were performed as in (g) on total cell lysates from C2C12 cells transfected with either R luc alone, R luc-3′HMGB1 or R luc-3′HMGB1-mut-miRBS. (h) Western blot was performed using an HuR antibody. This blot is a representation of three independent experiments. (i) The levels of miR-1192 in each IP were determined and are plotted with the s.e.m. of three independent experiments. ***P<0.0001, **P<0.001 (Student’st-test). Figure 6: HuR binding to a U8 element within HuRBS is sufficient to prevent the miR-1192-mediated inhibition of HMGB1 translation. ( a ) Schematic representation of the HuRBS and the seed element of miR-1192 (miR-1192 BS). ( b ) Diagram illustrating the bioinformatic approach used to predict miR-1192 as a putative miRNA targeting HMGB1 3′UTR. Shown here are complementarities of miR-1192 with HMGB1 3′UTR. ( c ) Schematic diagrams of luciferase constructs. ( d – g ) Effects of HuR, miRNAs, antagomirs and mimics. Error bars represent s.e.m of three independent experiments. *** P <0.0001, ** P <0.001, * P <0.05 (Student’s t -test). The amount of reporter RNA expressed in cells was determined by qPCR and used to normalize R Luc activities for each treatment. ( d ) Exponentially growing C2C12 cells were treated with siCtr or siHuR and 24 h later luciferase constructs were introduced. Luciferase activity of R Luc construct was considered as 100%. ( e ) miR-1192 and miR-16 antagomirs were transfected in siHuR-treated C2C12 cells previously transfected either with R luc alone or R luc-3′HMGB1. ( f ) Upper panel: schematic representation of the Mimic miR-1192 and Mimic mutant miR-1192. The asterisk (*) indicates the a – c mutation in the Mimic mutant miR-1192. Lower panel: HeLa cells were transfected with Mimic miR-1192 or Mimic mutant miR-1192 and 24 h later luciferase constructs were transfected. The luciferase activity of the mock-treated cells was set as reference. ( g ) Immunoprecipitation experiments were performed using a monoclonal HuR antibody, or IgG as a control, on total cell lysates from exponentially growing C2C12 cells. RNA was isolated from the immunoprecipitate, and quantitative RT–PCR was performed using primers specific to miR-1192, miR-16 and U6 RNAs. The levels of miR-1192 and U6 RNAs in each IP were normalized against the level of miR-16. Error bars represent s.e.m of three independent experiments. T -test was used for statistical analysis. ( h , i ) Immunoprecipitation experiments were performed as in ( g ) on total cell lysates from C2C12 cells transfected with either R luc alone, R luc-3′HMGB1 or R luc-3′HMGB1-mut-miRBS. ( h ) Western blot was performed using an HuR antibody. This blot is a representation of three independent experiments. ( i ) The levels of miR-1192 in each IP were determined and are plotted with the s.e.m. of three independent experiments. *** P <0.0001, ** P <0.001 (Student’s t -test). Full size image We first determined the impact of the miRBS and HuRBS on the translation of a reporter mRNA containing the HMGB1 3′UTR. For these experiments, we used a Renilla luciferase (R Luc) reporter containing either a wt (R Luc-3′HMGB1) or a mutated 3′UTR with mutations in the seed element of miR-1192 (R Luc-3′HMGB1-mut-miRBS), or the HuRBS (R Luc-3′HMGB1-mut-HuRBS) ( Fig. 6c ). Of note, as all the 15 Us of HuRBS were mutated in R Luc-3′HMGB1-mut-HuRBS, this reporter should be unable to recruit both HuR and miR-1192 to the HMGB1 -3′UTR. We transfected each one of the constructs in C2C12 cells depleted or not of HuR and measured luciferase activity [34] in comparison to the baseline activity of R Luc alone ( Fig. 6d ). In cells expressing endogenous HuR, the luciferase activity of R Luc-3′HMGB1 was >60% higher than R Luc alone ( Fig. 6d ). Mutating the HuRBS (R Luc-3′HMGB1-mut-HuRBS) prevented this increase, confirming that the binding of HuR to the HMGB1 -3′UTR actively promotes translation. Mutating the seed element of miR-1192 (R Luc-3′HMGB1-mut-miRBS), however, did not prevent the translation increase mediated by the HMGB1 -3′UTR. Indeed, REMSA experiments demonstrated that HuR can bind to the HuRBS despite mutations in miR-1192 seed element ( Supplementary Fig. S7 ). These results clearly indicate that the recruitment of HuR to the HuRBS is sufficient to promote the translation of HMGB1 in muscle cells. As the inhibition of HMGB1 translation occurs only in cells depleted of HuR ( Fig. 4 ), we repeated the experiments described above in HuR-knockdown C2C12 cells. We observed that the R Luc-3′HMGB1 reporter, unlike the R Luc-3′HMGB1-mut-miRBS or R Luc-3′HMGB1-mut-HuRBS constructs, displayed ~50% decrease in luciferase activity when compared with its control R Luc counterpart ( Fig. 6d ). Additionally, silencing miR-1192 by a miRNA silencer (antagomir Anti-miR-1192) abrogated the decrease in the luciferase activity mediated by the HMGB1 -3′UTR. No such effect was, however, seen in cells treated with a control antagomir against miR-16 (Anti-miR-16) ( Fig. 6e and Supplementary Fig. S8a ). Importantly, the concentration of antagomir used in these experiments did not affect the viability of C2C12 cells [35] , [36] , [37] and the steady state levels of endogenous HMGB1 mRNA ( Supplementary Fig. S8b–d ). We next generated mimics of miR-1192 with or without an A-to-C mutation in its 5th nucleotide ( Fig. 6f ). In HeLa cells, which do not express endogenous miR-1192 ( Supplementary Fig. S6 ), the mimic miR-1192 reduced the luciferase activity of R Luc-3′HMGB1 by ~50%. The mutant miR-1192 mimic, however, had no effect on this activity ( Fig. 6f ). The luciferase activity of the R Luc-3′HMGB1-mut-miRBS was not affected by the Mimic miR-1192, indicating that inhibition of R Luc-3′HMGB1 translation occurs via a direct binding to the miRBS. Collectively, these results demonstrate that in muscle cells, miR-1192 directly inhibits the translation of HMGB1 mRNA via the miRBS element, but this effect is overcome by the binding of HuR to its HuRBS. Our IP combined to miRNA microarray data ( Supplementary Table S2 ), which were validated by performing IP/RT–qPCR experiments ( Fig. 6g ) indicated that HuR and miR-1192 can coexist in the same complex in C2C12 cells. To determine whether this complex is indeed assembled on the HMGB1 -3′UTR, we performed the same IP/RT–qPCR experiment on C2C12 cells expressing either R Luc alone, R Luc-3 ′ HMGB1 or the R Luc-3 ′ HMGB1-mut-miRBS mRNAs. We observed that the level of miR-1192 in the HuR complex was fivefold greater in cells expressing the R Luc-3 ′ HMGB1 mRNA when compared with cells expressing mRNAs deficient in their ability to bind miR-1192 ( R Luc or R Luc-3 ′ HMGB1-mut-miRBS ) ( Fig. 6h,i ). Therefore, these observations clearly indicate that HuR and miR-1192 can bind simultaneously the 3′UTR of HMGB1 mRNA. We next verified mechanistically how HuR could negate the ability of miR-1192 to repress the translation of the HMGB1 mRNA. miRNAs are known to translationally repress mRNAs via the recruitment of the Ago2, a component of the RNA-induced silencing complex (RISC) [38] . We thus verified if HuR prevents the miR-1192-mediated recruitment of Ago2 to the HMGB1-miRBS. Our data indicate that although both HuR and miR-1192 simultaneously bind to the HMGB1 mRNA 3′UTR, the association of Ago2 to both miR-1192 and the HMGB1 mRNA is increased when HuR is depleted from C2C12 cells ( Fig. 7 ). These experiments, therefore, indicate that HuR prevents the miR-1192-mediated translational repression of the HMGB1 mRNA by interfering with the recruitment of Ago2. 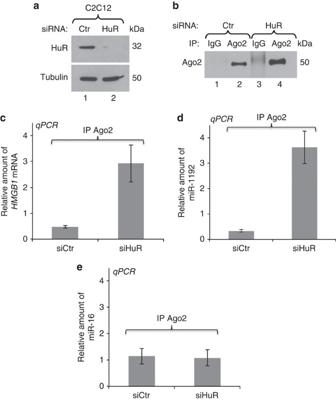Figure 7: HuR binding to the HuRBS prevents the recruitment of Ago2 to theHMGB1mRNA. (a) Western blot analysis was performed using antibodies against HuR and α-tubulin as a loading control on total cell extracts obtained from exponentially growing C2C12 cells treated with a control (Ctr) or HuR specific (siHuR) siRNA. (b) Immunoprecipitation experiments were performed using a monoclonal Ago2 antibody, or anti-IgG antibody as a control, on the total cell lysates described in (a). The immunoprecipitation of Ago2 was then assessed by western blotting using an anti-Ago2 antibody. (c–e) RNA was isolated from the immunoprecipitate described above, and quantitative RT–PCR was performed using primers specific to (c) HMGB1 (d) miR-1192 (e) miR-16. The levels ofHMGB1mRNA, miR-1192 and miR-16 in each IP, relative to those in the IgG IP, were respectively normalized against theGAPDHmRNA and U6 levels. Error bars represent s.e.m of three independent experiments. Figure 7: HuR binding to the HuRBS prevents the recruitment of Ago2 to the HMGB1 mRNA. ( a ) Western blot analysis was performed using antibodies against HuR and α-tubulin as a loading control on total cell extracts obtained from exponentially growing C2C12 cells treated with a control (Ctr) or HuR specific (siHuR) siRNA. ( b ) Immunoprecipitation experiments were performed using a monoclonal Ago2 antibody, or anti-IgG antibody as a control, on the total cell lysates described in ( a ). The immunoprecipitation of Ago2 was then assessed by western blotting using an anti-Ago2 antibody. ( c – e ) RNA was isolated from the immunoprecipitate described above, and quantitative RT–PCR was performed using primers specific to ( c ) HMGB1 ( d ) miR-1192 ( e ) miR-16. The levels of HMGB1 mRNA, miR-1192 and miR-16 in each IP, relative to those in the IgG IP, were respectively normalized against the GAPDH mRNA and U6 levels. Error bars represent s.e.m of three independent experiments. Full size image Our data show that HMGB1 is one of the mRNA targets through which HuR promotes myogenesis. Specifically, the results outlined in Fig. 6 suggest that HuR-depleted muscle cells fail to enter myogenesis because in the absence of HuR, miR-1192 inhibits HMGB1 translation. Hence, silencing miR-1192 should rescue HMGB1 expression in HuR-depleted muscle cells and should also re-establish their myogenic potential. Our experiments showed that silencing miR-1192 but not miR-16 prevented the inhibition of HMGB1 translation in HuR-depleted C2C12 cells ( Fig. 8a,b and Supplementary Fig. S9a ). In the presence of endogenous HuR, however, Anti-miR-1192 had no effect on HMGB1 translation ( Fig. 8a,b and Supplementary Fig. S9a ). This result was further confirmed by the fact that while the depletion of HuR shifted the distribution of HMGB1 mRNA towards lighter polysome fractions ( Fig. 4f ), silencing miR-1192 reversed this effect ( Supplementary Fig. S9b ). Next, we assessed whether the Anti-miR-1192-mediated rescue of HMGB1 translation is sufficient to promote the myogenic potential of HuR-knockdown cells. Indeed, silencing miR-1192 but not miR-16 re-established the myogenic potential of HuR-depleted cells ( Fig. 8c,d ) and the expression levels of My-HC, myoglobin and myogenin ( Fig. 8e ). 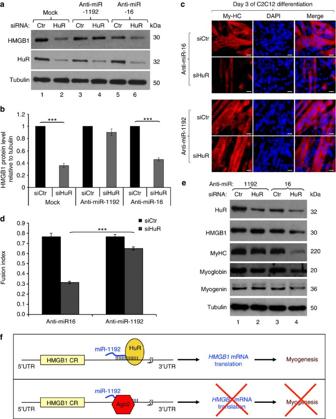Figure 8: Silencing miR-1192 reestablishes HMGB1 translation and rescues the myogenic potential of HuR-depleted muscle cells. (a) Exponentially growing C2C12 were treated with siCtr or siHuR and were transfected 5 h later with antagomirs to miR-1192 or miR-16. Extracts from these cells were harvested and used for western blotting with anti-HMGB1, -HuR and -α-tubulin antibodies. (b) The expression level of HMGB1 protein relative to α-tubulin. Error bars represent s.e.m. of three independent experiments. ***P<0.0001 (student’st-test). (c) C2C12 treated as in (a) were grown to confluency, induced to differentiate for three days and stained with anti-My-HC antibody and DAPI. Scale bars, 20 μm. The images shown are representative fields for each cell treatment from three independent experiments. (d) Fusion index of cells in (c). Error bars represent s.e.m. of three independent experiments. ***P<0.0001 (student’st-test). (e) Total extracts from cells treated as described above were blotted and probed with antibodies against HuR, HMGB1, My-HC, myoglobin, myogenin and α-tubulin. A representative blot of two independent experiments is shown. (f) Schematic model illustrating how HuR promotes the myogenesis in undifferentiated muscle cells. HuR recognizes an U8element in theHMGB1-3′UTR adjacent to the seed element of miR-1192, and promotes HMGB1 translation and myogenesis. HuR mediates this effect even if miR-1192 is bound to its seed element (upper panel). In the absence of HuR, however, miR-1192 recruits Ago2 thus inhibiting HMGB1 translation and preventing myogenesis (lower panel). Figure 8: Silencing miR-1192 reestablishes HMGB1 translation and rescues the myogenic potential of HuR-depleted muscle cells. ( a ) Exponentially growing C2C12 were treated with siCtr or siHuR and were transfected 5 h later with antagomirs to miR-1192 or miR-16. Extracts from these cells were harvested and used for western blotting with anti-HMGB1, -HuR and -α-tubulin antibodies. ( b ) The expression level of HMGB1 protein relative to α-tubulin. Error bars represent s.e.m. of three independent experiments. *** P <0.0001 (student’s t -test). ( c ) C2C12 treated as in (a) were grown to confluency, induced to differentiate for three days and stained with anti-My-HC antibody and DAPI. Scale bars, 20 μm. The images shown are representative fields for each cell treatment from three independent experiments. ( d ) Fusion index of cells in ( c ). Error bars represent s.e.m. of three independent experiments. *** P <0.0001 (student’s t -test). ( e ) Total extracts from cells treated as described above were blotted and probed with antibodies against HuR, HMGB1, My-HC, myoglobin, myogenin and α-tubulin. A representative blot of two independent experiments is shown. ( f ) Schematic model illustrating how HuR promotes the myogenesis in undifferentiated muscle cells. HuR recognizes an U 8 element in the HMGB1 -3′UTR adjacent to the seed element of miR-1192, and promotes HMGB1 translation and myogenesis. HuR mediates this effect even if miR-1192 is bound to its seed element (upper panel). In the absence of HuR, however, miR-1192 recruits Ago2 thus inhibiting HMGB1 translation and preventing myogenesis (lower panel). Full size image It was previously shown that miRNAs such as miR-519 and miR-16 inhibit HuR expression in various cell lines [39] , [40] , [41] . However, as HuR levels does not significantly change during the early steps of myogenesis in vitro [16] , [17] , [42] and increase during muscle regeneration in vivo [30] ( Supplementary Fig. S10 ), miRNA-mediated modulation of HuR expression in muscle cells seems to be ineffective in these conditions. Our experiments show that while the expression level of miR-16 increases during myogenesis both in vitro and in vivo ( Supplementary Fig. S11a,b ), it is the depletion but not the increased expression of miR-16 that modestly reduces the expression level of HuR, with limited effects on HMGB1 as well as My-HC and myoglobin ( Fig. 8e ). In fact, a marked reduction of HMGB1 expression and the inhibition of myogenesis is observed only when HuR level is further reduced by small interfering RNA ( Fig. 8e ). These observations indicate that miR-1192 is active only when HuR level is below a critical threshold. All together, our data support a model whereby HuR helps undifferentiated muscle cells to enter myogenesis by supporting the translation of HMGB1 transcripts and preventing the action of Ago2/miR-1192 ( Fig. 8f ). In this study we show that HMGB1 is required for muscle fibre formation both in vitro and in vivo and uncover a novel mechanism by which muscle cells modulate HMGB1 expression. A general reduction in skeletal muscle tissues was previously observed in Hmgb1 −/− mice, among several other defects [24] . Here we show that a precise level of HMGB1 expression is required for proper muscle fibre formation, as a 50% reduction in HMGB1 expression in embryos significantly decreases the efficiency of myogenesis. Thus, a tight control of HMGB1 expression levels appears essential for myogenesis. More than a decade ago, it was discovered that HMGB1 mRNA harbours a long 3′UTR with U-rich elements [43] , [44] , [45] suggesting that posttranscriptional events could regulate HMGB1 expression. Surprisingly, this possibility was never explored. Our data clearly establish that a posttranscriptional mechanism, via HuR, has a key role in promoting HMGB1 expression in muscle cells. HuR, one of the well known posttranscriptional regulators, affects the expression of its target mRNAs by binding to specific U-rich elements in their 3′UTRs [14] , [15] . We show that the 3′UTR of HMGB1 mRNA harbours such an element, the HuRBS, through which HuR promotes the translation of HMGB1 mRNA. In the absence of HuR, however, the microRNA miR-1192 is able to inhibit the expression of HMGB1. To our knowledge, this is the first report of the impact of a miRNA on HMGB1 expression. Incidentally, this is also the first report on the biological activity of miR-1192. Using several different techniques including miRNA microarray analysis, RT–qPCR with specific primers for miR-1192, and the sequencing of the PCR product that was generated by these primers, our data indicate that miR-1192 is expressed in muscle cells. Previous reports using RNA sequencing (RNA-seq), however, have failed to detect miR-1192 in the whole mouse embryo and muscle tissues [46] , [47] . As demonstrated by several recent studies [48] , [49] , technical biases during capture and preparation of the small RNA library has an impact on detection of small RNA molecules. Despite potential technical differences in methods used to precisely quantify the expression level of miR-1192 in muscle cells, our data clearly show that this miRNA is expressed in muscle cells and is functionally relevant in modulating HMGB1 expression. As HuR, HMGB1 and miR-1192 are highly expressed in muscle cells and during muscle regeneration [30] ( Supplementary Figs S10 and S11 ) and both HuR and miR-1192 can simultaneously associate with the HMGB1 -3′UTR, our data support a model whereby the binding of HuR to its HuRBS is sufficient to prevent miR-1192-mediated inhibition. Interestingly, the association of miR-1192 with Ago2, a key player in the RISC complex [38] , [50] , is dramatically enhanced in muscle cells depleted of HuR. This suggests that HuR prevents the action of miR-1192 by interfering with the recruitment of Ago2 to the HMGB1 3′UTR. These data are consistent with previous observations showing that HuR promotes the translation of target messages by preventing the assembly of an active RISC complex on the Let-7 miRNA seed element [51] even if its binding site is far away from the miRNA seed element. Therefore, these observations with our data suggest that HuR promotes the translation of target mRNAs by interfering with the formation of an active RISC complex regardless of the distance of its binding site from the seed element. This mechanism of action is different from the one described for the dead end 1 protein, another RBP, which promotes translation of the cyclin-kinase inhibitor p27 cip by preventing the recruitment of miR-221/222 to their seed elements [52] . Therefore, our findings not only add another example to the few studies on the cross talk between RNA-binding proteins and miRNAs, but also uncover a novel way by which cells, via proteins such as HuR, control miRNA-mediated effects. Our data demonstrate that via such a mechanism HuR induces the translation of HMGB1, which in turn promotes the entry of muscle cells into myogenesis. By linking the interplay between HuR and miR-1192 to the translation modulation of HMGB1, we found a posttranscriptional mechanism that controls the expression of the main ‘alarmin’ in the organism [53] , [54] . HMGB1 is a damage-associated molecular pattern molecule that upon severe injury activates the innate immune system to recognize tissue damage and initiate reparative responses [55] , [56] . Typically, the increase in HMGB1 levels in stressed or activated inflammatory cells precedes the upregulation of HMGB1 transcript levels by several hours [56] . Our results suggest that posttranscriptional events might be responsible for this increase, as the HMGB1 mRNAs are both abundant [43] , [44] and stable ( Supplementary Fig. S2 ). Therefore, our study may open the door to new strategies to manipulate HMGB1 levels under various conditions. Such a strategy could help promote the beneficial effects of HMGB1 (for example, the activation of muscle regeneration and wound healing) while limiting/preventing the deleterious outcomes of its overproduction during life-threatening assaults (for example, ischaemia, burn, infection or sepsis). Plasmid construction The pCMV-SPORT6 plasmid containing the full-length HMGB1 cDNA (accession number: BC008565) was purchased from Open Biosystems (catalogue number: MMM1013-64094). pRL-luc-3′HMGB1-mut-miRBS was generated by Norclone Biotech Laboratories, Kingston, ON, Canada. The full-length 3′UTR of mouse HMGB1 was subcloned into a pRL-SV40 vector (Promega) by performing PCR amplification using the following primers: forward 5′-TTG GTT CTA GCG CAG TTT TT-3′ and reverse 5′-TCA TCC AGG ACT CAT GTT CAG-3′. The pRL-SV40 vector was digested by Xba1 restriction enzyme (New England Biolabs), followed by a treatment with the T4 DNA polymerase, and then dephosphorylated. The PCR insert was ligated into the plasmid using the Quick Ligase enzyme (Promega) according to the manufacturer’s instructions. pRL-luc-3′HMGB1-mutHuRBS was generated using a specific primer containing the mutations and Quickchange site-directed mutagenesis kit (Stratagene). The MISSION short hairpin RNA (shRNA) plasmid (siHMGB1; Sigma-Aldrich) was used to knock down HMGB1. MISSION pLKO.1-puro vector encoding scrambled shRNA (siCtr; SHC001) was used as a control. Cell culture and transfection C2C12 muscle cells (ATCC) were grown in media containing 20% fetal bovine serum (Invitrogen) in DMEM (Dulbecco’s modified eagle medium from Invitrogen). In order to induce muscle cell differentiation, cells were switched to a media containing DMEM, 2% horse serum, penicillin/streptomycin antibiotics (Invitrogen), and 50 mM HEPES, pH 7.4 (Invitrogen) when their confluency reached 100% (refs 17 , 42 ). Hmgb1 +/+ and Hmgb1 −/− mouse embryonic fibroblasts (MEFs) (HMGBiotech, Milan, Italy) were cultured in DMEM supplemented with penicillin/streptomycin and 10% fetal bovine serum (Sigma-Aldrich). Transfections with small interfering RNAs specific for HuR or plasmids were performed using Lipofectamine and Plus reagents (Invitrogen) or jetPEI (Polyplus Transfection) according to the manufacturer’s instructions. The same transfection protocol was used to treat C2C12 cells with 200 nM miR-1192 or miR-16 antagomirs (Dharmacon). HMGB1 rescue experiments Transient transfection of C2C12 cells was carried out using jetPEI (Polyplus Transfection), as recommended by the manufacturer. Briefly, C2C12 cells were transfected with the MISSION shRNA plasmid (Sigma-Aldrich) to knock down HMGB1 or with the MISSION pLKO.1-puro vector encoding a scrambled shRNA (SHC001) as a control. Forty-eight hours post-transfection, the cells were switched to differentiation media and cultured for additional 48 h in the absence or presence of recombinant HMGB1 (400 nM). Preparation of cell extracts and immunoblotting Total cell extracts were prepared by incubating undifferentiated or differentiated C2C12 cells on ice for 15 min with lysis buffer (50 mM HEPES pH 7.0, 150 mM NaCl, 10% glycerol, 1% Triton, 10 mM pyrophosphate sodium, 100 mM NaF, 1 mM EGTA, 1.5 mM MgCl 2 , 1 × protease inhibitor (Roche), 0.1 M orthovanadate, 0.2 M PMSF), then centrifuge at 12,000 g at 4 °C and the supernatant was kept [17] . The extracts were run on an SDS–PAGE and transferred to nitrocellulose membranes (Bio-Rad). The samples were analysed by western blotting [57] with antibodies against HuR (3A2,1:10,000) [57] , HMGB1 (Abcam,1:1,000), My-HC (MY32;Sigma,1:1,000), Myogenin (F5D, Developmental studies Hybridoma Bank, 1:250), α-tubulin (Developmental studies Hybridoma Bank, 1:1,000), hnRNPA1 (Cell Signalling, 1:1,000) [22] , β-actin (Sigma,1:500), myoglobin (DAKO, 1:500) and Ago2 (Cell Signalling,1:1000). Full blots are provided in Supplementary Fig. S12 . Immunofluorescence IF was performed using undifferentiated or differentiated C2C12 cells that were grown to sub-confluency in DMEM (Dulbecco’s modified eagle medium from Invitrogen) [17] . After the appropriate experimental treatments, cells were rinsed twice in phosphate-buffered saline (PBS), fixed in 3% phosphate-buffered paraformaldehyde (Sigma) and permeabilized in 0.5% PBS-goat serum with Triton. After permeabilization, cells were incubated with primary antibodies against My-HC (MF-20, developmental studies Hybridoma Bank, 1:1,000), HuR (3A2,1:1,000) or HMGB1 (Abcam,1:1,000)) for 1 h at room temperature and then incubated with goat anti-mouse or anti-rabbit secondary antibodies conjugated with Rhodamine ( red ) or FITC ( gree n) from Molecular Probes (Eugene, OR). To visualize the nucleus, cells were stained with DAPI (Molecular Probes). Microscopic analyses were performed using an AXIOVERT 200 M (Zeiss). β-Galactosidase staining MLC1/3F-nlacZ homozygous transgenic mice [25] were mated with Hmgb1 +/− heterozygotes. Pregnant females were killed by cervical dislocation at E10.5. Embryos were isolated in PBS, fixed for 2 h in 4% paraformaldehyde pH 7.4 at 4 °C, washed in PBS for 20 min and equilibrated in 20% sucrose PBS. Fixed embryos were then stained for 1 h at 37 °C in 1 mg ml −1 X-gal solution of PBS, also containing 5 mM K 4 Fe(CN) 6 , 5 mM K 3 Fe(CN) 6 , 2 mM MgCl 2 , 0.2% NP-40 PBS. Hmgb1 +/− embryos were identified by PCR analysis of yolk sac DNA using the following primers: HMGB1for 5′-GCA GGC TTC GTT GTT TTC ATA CAG-3′ and HMGB1rev 5′-TCA AAG AGT AAT ACT GCC ACC TTC-3′ for the wt allele; NEOfor 5′-TGG TTT GCA GTG TTC TGC CTA GC-3′ and NEOrev 5′-CCC AGT CAT AGC CGA ATA GCC-3′ for the targeted allele. These animal studies were approved by the San Raffaele University Animal Care Committee. Histology and morphometric analysis TA muscles were dissected from 1-year-old wild-type and Hmgb1 +/− mice and frozen in liquid nitrogen-cooled isopentane. Serial sections (8 μm thick) were stained with hematoxylin and eosin. Morphometric analyses were performed on sections of TA using ImageJ to determine the cross-sectional area of 900 fibres for each group. Fusion index Explants of presomitic mesoderm [58] were dissected from wt, Hmgb1 +/− and Hmgb1 −/− embryos at E9.5, plated on collagen-coated dishes and cultured for 4 days in DMEM supplemented with 20% FCS and 50 μg ml −1 gentamycin. On day 4, cultures were processed for immunoflorescence with an antibody specific for My-HC (MF-20, Developmental Studies Hybridoma Bank, 1:20 dilution). Fusion index was determined as the number of nuclei in sarcomeric myosin-expressing cells with more than two nuclei versus the total number of nuclei. Regeneration assay Muscle injury was performed on the TA of 3-month-old wt and Hmgb1 +/− mice by injecting 50 μl of 10 μM CTX (three animals per group). Mice were killed 3, 7 or 14 days after CTX injection, and the TA muscles were dissected and frozen in liquid N 2 –cooled isopentane. Ten-micrometre serial muscle sections were stained with hematoxylin and eosin. Alternatively, injury of C57BL/6 (Charles River) mouse muscles was performed by BaCl 2 injection in the TA muscle of 8-week old mice, under zolazepam/tiletamine anaesthesia [59] . These animal studies were approved by the San Raffaele University Animal Care Committee. RNA electromobility shift assays The HMGB1 cRNA probes were produced by in vitro transcription using a T7 RNA polymerase [60] . All HMGB1 probes (5′UTR and P1 to P12) were generated by PCR amplification using a forward primer fused to the T7 promoter as well as pCMV-HMGB1 expression vector as the template (see Supplementary Table S4 ). For smaller probes (P4-1 to P4-3), oligonucleotide sense and anti-sense were directly annealed and used for in vitro transcription. The RNA-binding assays were performed [22] by incubating either 10 μg total cell extracts or 300 ng purified recombinant protein (GST or GST-HuR) with 50,000 c.p.m. of 32 P-labelled cRNAs in a total volume of 20 μl EBMK buffer (25 mM HEPES pH 7.6, 1.5 mM KCl, 5 mM MgCl 2 , 75 mM NaCl, 6% sucrose and protease inhibitors) at RT for 15 min. For competition assays, 0.01 × , 0.1 × , 1 × , 10 × and 100 × excess unlabelled specific or unspecific transcripts were incubated with the TCE for 15 min at RT before the 32 P-labelled probes were added to the reaction. Two microlitres μl of a 50 mg ml −1 heparin sulphate stock solution was then added to the reaction for an additional 15 min at RT. In supershift experiments, 5 μg of a purified monoclonal anti-HuR antibody was then added to the reaction for an additional 15 min at RT. Samples were then loaded on a 4% polyacrylamide gel containing 0.05% NP-40. Quantitative RT–PCR One microgram of total RNA was reverse transcribed using the M-MuLV Reverse Transcriptase (New England Biolabs) according to the manufacturer’s protocol. A total of 1/80 dilution of cDNA was used to detect HMGB1 , GAPDH and R luc mRNAs using SsoFast EvaGreen Supermix (Bio-Rad). Expression of HMGB1 and R luc was standardized using GAPDH as a reference, and relative levels of expression were quantified by calculating 2 - ΔΔ C T is the difference in CT between target and reference. For miRNA detection, 200 ng of total RNA was reverse transcribed using the Universal cDNA synthesis kit (Exiqon) and the presence of miR-1192, miR-16 and U6 was assessed by qPCR using the SyBr Green Master Mix (Exiqon). Northern blot analysis and Actinomycin D pulse-chase experiments The extraction of total RNA was performed using Trizol reagent (Invitrogen) [22] . For the isolation of miRNAs, twice as much isopropanol was used in the RNA purification protocol. Northern blot analysis was performed using 10 μg total RNA [22] . After transferring to a Hybond-N membrane (Amersham) and UV-cross-linking, the blot was hybridized with probes specific for MyoD [17] , GAPDH [17] , 18S [61] , 5.8S [34] and HMGB1 mRNAs were generated using the PCR Purification Kit (GE Healthcare) with primers described below. The probes were radiolabelled with α− 32 P dCTP using Ready-to-Go DNA labelling beads (GE Healthcare) according to the manufacturer’s instructions. The stability of HMGB1 mRNA was assessed by the addition of the general transcriptional inhibitor actinomycin D (5 μg ml −1 ) [61] for the indicated periods of time. Total RNA was isolated from the cells after 0, 4, 6, 8, 10 and 12 h following ActD treatment using TRIzol reagent (Invitrogen), and analysed by northern blotting. Full blots are provided in Supplementary Fig S12 . For miRNA detection, 25 μg of total RNA was separated on a 12% denaturing urea polyacrylamide gel. RNA was subsequently transferred to a Hybond-N + membrane (Amersham Biosciences) and cross-linked to the membrane. Hybridization was carried out by using ULTRAHybOligo solution according to the manufacturer's instructions (Ambion). The probe sequences were complementary to the mature forms of miR-16 or U6 RNA and were labelled using StarFire system (Integrated DNA Technologies) according to the manufacturer’s protocol. Polysome fractionation Forty million myoblasts were grown and treated with small interfering RNAs as described above and polysome fractionation experiments were performed. Briefly, the cytoplasmic extracts obtained from lysed myoblast cells were centrifuged at 130 000 g for 2 h on a sucrose gradient (10–50% w/v) [62] , [63] . Polysomal (P) or non-polysomal (NP) fractions were pooled and RNA was extracted using Trizol LS (Invitrogen). RNA samples were then analysed on an agarose gel. The levels of HMGB1 and GAPDH mRNAs were determined using quantitative RT–PCR. Luciferase activity The activity of R Luc was measured using a Renilla luciferase assay system (Promega) with a luminometer following the manufacturer’s instructions. Fluorescence in situ hybridization The fluorescence in situ hybridization experiments were performed [29] using a DNA fragment of ~500 bp corresponding to the coding region of mouse HMGB1. The fragment was amplified by PCR using the following primers fused to either a T7 or T3 minimal promoter sequence: HMGB1 forward, 5′-AAA AAG CCG AGA GGC AAA AT-3′, and HMGB1 reverse, 5′-CTT TTT CGC TGC ATC AGG TT-3′. The PCR product was used as the template for in vitro transcription of the HMGB1 probe needed for fluorescence in situ hybridization. The anti-sense (T3) and sense (T7) probes were prepared using digoxigenin-RNA labelling mix from Roche Diagnostics. The RNA probes were quantified, denatured and incubated with permeabilized cells at 37 °C overnight in the hybridization buffer (50% formamide, 5 × SSC, 50 mM phosphate buffer, pH=7.4, 5 × Denhardt’s, 1 mM EDTA and 250 ng μl −1 of salmon sperm DNA). After the hybridization, the cells were used for IF to detect the HMGB1 mRNA and HuR protein [29] . Finally, the cells were incubated with secondary goat anti-rabbit antibody and anti-DIG antibody for IF. Preparation of mRNA complexes and analysis with RT–PCR TCE were prepared in lysis buffer (50 mM Tris, pH 8; 0.5% Triton X-100; 150 mM NaCl; complete protease inhibitor from Roche). Twenty-five microlitres of the anti-HuR (3A2) or IgG (Jackson Immunoresearch Laboratories) antibodies were incubated with 200 μl of pre-swelled protein A-Sepharose beads for 4 h at 4 °C. Alternatively, C2C12 cells depleted or not of HuR were incubated with an anti-Ago2 (Cell Signalling) or IgG control antibody. After three washes in lysis buffer, 1.5 mg of cell extract was added overnight at 4 °C. The final dilution of the antibodies during the incubation with lysates is 1/18. Beads were washed three times with cell lysis buffer, incubated with proteinase K and the RNA isolated by phenol/chloroform extraction followed by precipitation overnight at −20 °C with isopropanol [17] , [64] . Purified RNA was resuspended in 12 μl of water, and 2 μl was reverse transcribed using the M-MuLV Reverse Transcriptase (New England Biolabs) according to the manufacturer’s protocol. Association of HMGB1 and β -actin mRNAs with HuR as well as HMGB1 with Ago2 was defined using quantitative RT–PCR. Ten microlitres of purified RNA was reverse transcribed using the Universal cDNA synthesis kit (Exiqon) and the presence of miR-1192, miR-16 and U6 was assessed by qPCR. cDNA array analysis Microarray experiments were performed using mouse array, which contain 17,000 probe sets of known and unknown expressed sequence tags [65] . HuR was immunoprecipitated from exponentially growing C2C12 cells using an anti-HuR monoclonal antibody (3A2) and an anti-IgG monoclonal antibody as a negative control. The final dilution of the antibodies during the overnight incubation with lysates is 1/18. Then the samples were spun 5 min at-3,000 g and washed with TSE1 (0.1% SDS, 1% Triton X-100, 2 mM EDTA, 20 mM Tris-HCl pH: 8.1, 150 mM NaCl), TSE2 (0.1% SDS, 1% Triton X-100, 2 mM EDTA, 20 mM Tris-HCl pH: 8.1, 500 mM NaCl) and TSE3 (0.25 M, LiCl, 1% NP-40, 1% deoxycholate, 1 mM EDTA, 10 mM Tris-HCl pH: 8.1) buffers. The immunoprecipitate were then incubated for 30 min at 55 °C in 100 ml NT2 buffer (50 mM Tris pH:7.4, 150 mM NaCl, 1 mM MgCl 2 , 0.05% NP-40) with0.1% SDS and 30 mg proteinase K. The associated RNAs were extracted by adding ~15 ml of 2 M NaOAc pH: 4.0, 150μl of water saturated phenol and ~30 μl chloroform followed by 15 min incubation on ice. After spinning (12,000 g for 20 min) the aqueous phase is mixed with glycogen and isopropanol and incubated overnight at −20 °C. The isolated RNAs were then resuspended in water and hybridized on cDNA arrays. The data were processed using the Array Pro software (Media Cybernetics), then normalized by Z -score transformation [66] and used to calculate differences in signal intensities. Significant values were tested using a two-tailed Z -test and a P of ≤0.01. The data were calculated from two independent experiments. Subcellular fractionation Subcellular fractionation was performed using the PARIS kit (Ambion) (Austin, TX) according the manufacturer's instructions. An equal number of cells per sample were used. Biotin pull-down assay The P4 fragment of the 3′UTR of mouse HMGB1 was subcloned into a pGEM-Teasy vector (Promega) according to the manufacturer’s instructions by performing PCR amplification using the following primers: forward 5′-GCC ACT AAC CTT GCC TGG TA-3′ and reverse 5′-TCG TAT AAG CTG CAT CAG AGA CA-3′. The transcript is transcribed using the T7RiboMAX Express large scale RNA production system (Promega) according to the manufacturer’s instructions using the NotI digested PGEM-Teasy-P3P4 vector as a template. For preparing protein extracts, 30–40 millions of cells were washed with ice-cold PBS and resuspended in 1 ml of EBMK buffer (25 mM Hepes pH 7,6; 5 mM MgCl 2 ; 1,5 mM KCl; 75 mM NaCl; 175 mM sucrose) containing 0,5% NP-40, complete protease inhibitor without EDTA (Roche). Lysates were sonicated for 10 s 3 times at 200 W and cleared by centrifugation at 12,000 g for 15 min. The protein concentration was determined (Bio-Rad microassay) and 1 mg were used for each assay. Biotin pull-down assay is performed using Miltenyi Biotech mMACS streptavidin kit according to the manufacturer’s instructions. Primers used to prepare probes for northern blot analysis mHMGB1: For: 5′-GCA TCC TGG CTT ATC CAT TG-3′; rev: 5′-TGC TCT TTT CAG CCT TGA CC-3′ mGAPDH: For: 5′-AAG GTC ATC CCA GAG CTG AA-3′; rev: 5′-AGG AGA CAA CCT GGT CCT CA-3′ Statistical analyses The statistical analyses in this study were performed using the Graphpad Prism5 software to determine significance (two-tailed, Student’s t -test). Accession codes: Microarray data have been deposited in Gene Expression Omnibus under accession code GSE49857 . How to cite this article: Dormoy-Raclet, V. et al. HuR and miR-1192 regulate myogenesis by modulating the translation of HMGB1 mRNA. Nat. Commun. 4:2388 doi: 10.1038/ncomms3388 (2013).